Modular optimization of multi-gene pathways for fatty acids production inE. coli Microbial fatty acid-derived fuels have emerged as promising alternatives to petroleum-based transportation fuels. Here we report a modular engineering approach that systematically removed metabolic pathway bottlenecks and led to significant titre improvements in a multi-gene fatty acid metabolic pathway. On the basis of central pathway architecture, E. coli fatty acid biosynthesis was re-cast into three modules: the upstream acetyl coenzyme A formation module; the intermediary acetyl-CoA activation module; and the downstream fatty acid synthase module. Combinatorial optimization of transcriptional levels of these three modules led to the identification of conditions that balance the supply of acetyl-CoA and consumption of malonyl-CoA/ACP. Refining protein translation efficiency by customizing ribosome binding sites for both the upstream acetyl coenzyme A formation and fatty acid synthase modules enabled further production improvement. Fed-batch cultivation of the engineered strain resulted in a final fatty acid production of 8.6 g l −1 . The modular engineering strategies demonstrate a generalized approach to engineering cell factories for valuable metabolites production. Global energy demand, rising petroleum prices and environmental concerns have stimulated increased efforts to develop more sustainable and cost-effective fuels that could replace traditionally used fossil fuels. Exploitation of the diverse microbial pathways based on metabolic engineering and synthetic biology frameworks provides a promising solution to de novo synthesis of drop-in transportation fuels directly from microbial cells [1] . Among all the fuel molecules produced from living organisms, fatty acids and their derivatives have the highest volumetric energy density as most of the carbons in the long hydrocarbon chains are still in the reduction state [2] . With physicochemical properties closely resembling those of petroleum-based fuels, fatty acid-based fuels offer some unique advantages as compared with other fuel supplements (ethanol or butanol) such as lower hygroscopicity, miscibility with diesel fuels, lower downstream purification costs and compatibility with existing infrastructure [3] . Therefore, a number of fatty-acid-derived fuel molecules including free fatty acids [4] , alkane/alkene hydrocarbons [5] , [6] , fatty alcohols [7] , alkyl ketones [8] and triacylglyceride [9] have been produced from the fatty acid biosynthetic pathway. For instance, manipulation of precursor malonyl-CoA availability along with the expression of specific plant acyl-ACP thioesterases have resulted in fatty acid production at 2.5 g l −1 in E. coli [4] , [10] . A consolidated bioprocess combined fatty acid pathway with xylan-utilization pathway led to fatty acid ethyl esters production at 11.8 mg l −1 (ref. 11 ). Using ionic liquid-pretreated switch grass as substrate, the same group has achieved fatty acid ethyl esters production at 70 mg l −1 (ref. 12 ). Engineering the reversal of β-oxidation pathway coupled with endogenous dehydrogenases and thioesterases have been used to produce fatty acids at 6.9 g l −1 in E. coli [7] . Despite these exciting achievements, there exists a pressing need to develop economically viable processes with high yield and productivity. However, engineering microbial overproduction phenotypes remains a daunting task as it usually involves the manipulation of a handful of precursor or rate-limiting pathways that are subjected to tight cellular regulation. For example, precursor flux improvement by overexpression of heterologous pathways may not be accommodated by downstream pathways; accumulated or depleted intermediates may compromise cell viability and pathway productivity [13] . As an attempt to address these issues, combinatorial transcriptional engineering coupled with efficient gene assembly tools has offered tremendous opportunities for customized optimization of multi-gene pathways [14] . Excellent examples include creation of yeast xylose pathways by promoter shuffling [15] , heterologous production of anticancer taxol precursors in E. coli [16] and rapid assembly and screening of multi-gene mutant pathway libraries in E. coli and yeast [17] , [18] . In the present work, we describe modular pathway engineering strategies to optimize a multi-gene pathway for fatty acid production in E. coli . By re-casting E. coli ’s central carbon metabolic network as a collection of distinct modules, we have assessed and eliminated pathway bottlenecks at both transcriptional and translational levels. Specifically, a total of 15 essential genes were selected and arranged into three modules to partition the complete fatty acid metabolic pathway into acetyl-CoA formation, acetyl-CoA activation and malonyl-ACP consumption pathways. Combinatorially tuning pathway expression by altering plasmid copy number led to balanced precursor distribution between the acetyl-CoA-producing pathway and acetyl-CoA/malonyl-CoA consumption pathways. Tuning translational efficiency by allocating customized ribosome binding sites (RBS) to both the precursor pathway and fatty acid synthase pathway enabled further fatty acid production improvement. Under controlled culture conditions, the engineered strains produced up to 8.6 g l −1 fatty acids with the highest productivity (0.124 g l −1 h −1 ) reported to date. The present work highlights the importance of systematic optimization of multi-gene pathways to enable an efficient microbial production of fuels. Engineering the fatty acid biosynthetic pathway in E. coli A common metabolic engineering strategy to improve product yield is to overexpress bottleneck enzymes and knockout competing pathways to increase carbon flux towards a pathway of interest. As an initial attempt to increase fatty acid production in E. coli , we sought to delete the fatty acyl-CoA synthetase ( fadD ) pathway with two aims: (i) block the fatty acid degradation pathway and (ii) relieve the allosteric inhibition of acetyl-CoA carboxylase by the accumulated fatty acyl-CoAs [19] . However, the engineered strain yielded only a minor increase in fatty acid production ( Fig. 1b ), suggesting that other rate-limiting factors needed to be addressed. Coupled with the overexpression of the four subunit acetyl-CoA caboxylase (ACC encoded by accABCD ) from E. coli to increase carbon flux towards the precursor malonyl-CoA, the modified strain demonstrated a three-fold increase in fatty acid production ( Fig. 1b ). Indeed, improved cellular concentration of malonyl-CoA by expression of E. coli or heterologous ACC has proven to be an effective approach to increase the production titre of a range of malonyl-CoA-derived compounds including flavonoids [20] , polyketides [21] and fatty acids [4] , [22] . 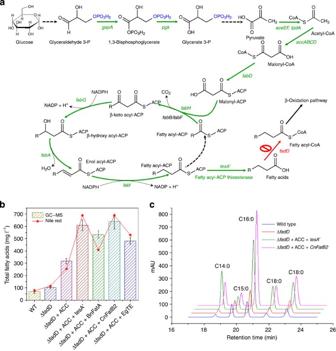Figure 1: EngineeringE. colifatty acid metabolic pathway. (a)E. colifatty acid biosynthetic pathway. Overexpression targets are shown in green and knockout targets in red. Dash arrows represent multiple reaction steps.accABCD, acetyl-CoA carboxylase;fabD, malonyl-CoA-ACP transacylase;fabH, β-ketoacyl-ACP synthase III;fabB, β-ketoacyl-ACP synthase I;fabF, β-ketoacyl-ACP synthase II;fabG, β-ketoacyl-ACP reductase;fabA, β-hydroxy acyl-ACP dehydrase;fabI, enol acyl-ACP reductase;tesA′, truncated multifunctional fatty acyl-CoA thioesterase; andfadD, fatty acyl-CoA synthetase. (b) Fatty acid production inE. coliBL21ΔfadDexpressing four subunits of acetyl-CoA carboxylase and plant fatty acyl-ACP thioesterase quantified by GC–MS and Nile red assay. Bars show fatty acid production analysed by GC–MS; red star shows fatty acid production analysed by Nile red assay. BnFatA,B. napusfatty acyl-ACP thioesterase (Gene ID: X73850.1); CnFatB2,C. nuciferafatty acyl-ACP thioesterase (Gene ID: JF338904.1); EGTE,E. guineensisfatty acyl-ACP thioesterase (Gene ID: AF110462.1). All experiments were performed in triplicate and error bars show s.d. with 95% CI. (c) High-performance liquid chromatography (HPLC) profile of fatty acids phenacyl esters from engineered strains expressing different thioesterases. Figure 1: Engineering E. coli fatty acid metabolic pathway. ( a ) E. coli fatty acid biosynthetic pathway. Overexpression targets are shown in green and knockout targets in red. Dash arrows represent multiple reaction steps. accABCD , acetyl-CoA carboxylase; fabD , malonyl-CoA-ACP transacylase; fabH , β-ketoacyl-ACP synthase III; fabB , β-ketoacyl-ACP synthase I; fabF , β-ketoacyl-ACP synthase II; fabG , β-ketoacyl-ACP reductase; fabA , β-hydroxy acyl-ACP dehydrase; fabI , enol acyl-ACP reductase; tesA′ , truncated multifunctional fatty acyl-CoA thioesterase; and fadD , fatty acyl-CoA synthetase. ( b ) Fatty acid production in E. coli BL21Δ fadD expressing four subunits of acetyl-CoA carboxylase and plant fatty acyl-ACP thioesterase quantified by GC–MS and Nile red assay. Bars show fatty acid production analysed by GC–MS; red star shows fatty acid production analysed by Nile red assay. BnFatA, B. napus fatty acyl-ACP thioesterase (Gene ID: X73850.1); CnFatB2, C. nucifera fatty acyl-ACP thioesterase (Gene ID: JF338904.1); EGTE, E. guineensis fatty acyl-ACP thioesterase (Gene ID: AF110462.1). All experiments were performed in triplicate and error bars show s.d. with 95% CI. ( c ) High-performance liquid chromatography (HPLC) profile of fatty acids phenacyl esters from engineered strains expressing different thioesterases. Full size image Further steps to improve fatty acid production in E. coli include cytosolic expression of multifunctional fatty acyl-CoA synthetase ( tesA ′) [4] and plant-derived fatty acyl-ACP thioesterases [6] to alleviate the feedback inhibition of β-ketoacyl-ACP synthase by the accumulated fatty acyl-ACPs [23] . Crude fatty acids were extracted, derivatized and analysed by gas chromatography mass spectrometry (GC–MS) (a representative chromatographic profile can be found in Supplementary Fig. S1 ). Table 1 summarizes the major fatty acid methyl esters identified from the engineered cell culture. These were the methyl ester derivatives of myristic acid (C14:0), palmitoleic acid (C16:1ω7), palmitic acid (C16:0), vaccenic acid (C18:1ω7) and stearic acid (C18:0). By expressing a truncated tesA′ , the fatty acid production was increased by 90% compared with the parental strain ( Fig. 1b ). Expression of three different codon-optimized plant fatty acyl-ACP thioesterases ( BnFatA , CnFatB2 and EGTE ) led to the identfication of BnFatA as the best thioesterase to be expressed to further improve fatty acid production ( Fig. 1b ), albeit at moderate levels. Interestingly, we found that the fatty acid composition was dramatically changed as a result of expressing different fatty acyl-ACP thioesterases ( Fig. 1c ). Expressing the E. coli native thioesterase ( tesA′ ) shifted the fatty acid profile to medium chain myristic acid (C14:0); whereas expressing the Cocos nucifera fatty acyl-ACP thioesterase ( CnFatB2 ) shifted the major fatty acids to palmitic acid (C16:0) compared with the parental strain. Detailed fatty acid composition can be found in Supplementary Fig. S2 . As an attempt to develop a rapid fatty acid detection protocol, we also compared the quantification results obtained from the GC–MS analysis with those obtained from a Nile red assay. The Nile red data shows a very strong correlation with the GC–MS data ( R 2 =0.925, Fig. 1b and Supplementary Fig. S3 ), indicating such an assay could potentially be used as a high-throughput screen for identifying the next generation of fatty acid-overproducing mutants. Table 1 GC–MS profile of fatty acids methyl esters from metabolically engineered E. coli . Full size table In our previous work [20] , using a constraint-based flux balance model, we identified gene targets whose overexpression and deletion led to a four-fold increase in cellular acetyl-CoA/malonyl-CoA levels. These targets included overexpression of glycolytic pathway enzymes such as glyceraldehyde-3-phosphate dehydrogenase ( gapA ), phosphoglycerate kinase ( pgk ) and pyruvate dehydrogenase multi-enzyme complex ( aceEF and lpdA ) along with the expression of the ACC pathway. Besides these targets, we also investigated whether the E. coli fatty acid synthase multi-enzyme complex (encoded by fabA , fabD , fabG and fabI ) would increase the fatty acid production. Both glycolytic pathway and fatty acid synthase pathway were assembled onto either a high copy number plasmid or a medium copy number plasmid. Overexpression of either glycolytic pathway enzymes or enzymes from the fatty acid biosynthetic pathway did improve the production titres in both the tesA′ and CnFatB2 expression strains ( Supplementary Figs S4 and S5 ). However, coexpression of glycolytic pathway enzymes and fatty acid biosynthetic enzymes led to a suboptimal production phenotype ( Supplementary Figs S4 and S5 ), indicating a metabolic imbalance between the supply of acetyl-CoA and the consumption of malonyl-CoA. These results demonstrate that the relative levels of intermediate metabolites can dramatically affect the production potential of an engineered pathway, possibly due to the buildup of toxic intermediates, which would elicit stress responses that are detrimental to cell growth [24] , [25] . Modular pathway optimization improves fatty acid production Considering the large subsets of engineering targets and their combinations, it is impractical to exhaustively explore the entire metabolic space for engineering fatty acid overproduction phenotypes. To circumvent these limitations, we took a multivariate modular approach to optimize the metabolic balance between acetyl-CoA-producing pathways and malonyl-CoA-consuming pathways. On the basis of the central metabolic pathway architectures ( Fig. 1a ), the E. coli fatty acid biosynthetic pathway was decomposed into three modules, (i) GLY module: upstream glycolysis module encoded by pgk , gapA , aceE , aceF and lpdA ; (ii) ACA module: intermediary acetyl-CoA activation module encoded by fabD , accA , accB , accC and accD ; and (iii) FAS module: downstream fatty acid biosynthetic module encoded by CnfatB2 , fabA , fabH , fabG and fabI ( Fig. 2a ). Using a recently developed synthetic biology platform that streamlines the process of gene assembly and pathway construction [26] , the GLY, ACA and FAS modules were successfully expressed on the five compatible ePathBrick vectors ( Supplementary Table S1 ), with varying promoter strength, plasmid copy number and antibiotic resistance marker. 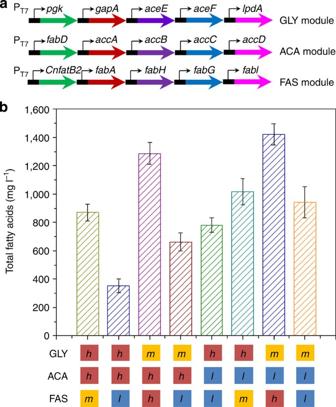Figure 2: Transcriptional fine tuning by varying plasmid copy number. (a) Three modules in theE. colifatty acid biosynthetic pathway: GLY, ACA and FAS module. (b) Optimization of fatty acid production through balancing the expression of GLY, ACA and FAS modules. Three modules were expressed either on (h) high copy number plasmids (pETM6 or pRSM3), (m) medium copy number plasmid (pCDM4) or (l) low copy number plasmids (pACM4 or pCOM4). All experiments were performed in triplicate and error bars show s.d. with 95% CI. Figure 2: Transcriptional fine tuning by varying plasmid copy number. ( a ) Three modules in the E. coli fatty acid biosynthetic pathway: GLY, ACA and FAS module. ( b ) Optimization of fatty acid production through balancing the expression of GLY, ACA and FAS modules. Three modules were expressed either on ( h ) high copy number plasmids (pETM6 or pRSM3), ( m ) medium copy number plasmid (pCDM4) or ( l ) low copy number plasmids (pACM4 or pCOM4). All experiments were performed in triplicate and error bars show s.d. with 95% CI. Full size image The upstream module (GLY) comprising the glycolysis pathway provides the acetyl-CoA source necessary for fatty acid production; whereas the downstream module (FAS) comprising the fatty acid chain initiation/elongation/termination steps provides a malonyl-ACP sink for fatty acid production. The two modules were linked and regulated through the intermediary ACA module to channel carbon flux from acetyl-CoA to malonyl-ACP ( Figs 1a and 2a ) and enable fatty acid production. By expressing these three modules either on high ( h ), medium ( m ) or low ( l ) copy number plasmids ( Fig. 2b ), we have systematically identified conditions that optimally balance the expression of acetyl-CoA-producing pathways (GLY module) and malonyl-ACP-consuming pathways (FAS module). For example, the expression of ACA module accompanied by the expression of FAS module from low copy number plasmids ( h ACA- l FAS and l ACA- l FAS) led to a relatively low fatty acid production, possibly due to the accumulated toxic malonyl-CoA/ACP intermediates that cannot be accommodated by the capacity of the downstream FAS module ( Fig. 2b ). Similarly, the lower production in the h GLY- h ACA and h GLY- l ACA strains can be attributed to the accumulated acetyl-CoA that is detrimental to cell growth [25] . Interestingly, the expression of the ACA module from low copy number plasmids led to higher fatty acid production compared with expression of the ACA module from high copy number plasmids, indicating that lower expression of ACA was sufficient to convert acetyl-CoA to malonyl-ACP. By expressing the acetyl-CoA source pathways on medium copy number plasmids and expressing the malonyl-ACP sink pathways on high copy number plasmids, we were able to minimize the accumulation of toxic acetyl-CoA/malonyl-ACP intermediates, and achieved a total fatty acid production of 1.42 g l −1 from the optimal strain ( m GLY- l ACA- h FAS). These results indicated that balancing metabolic pathway precursors was an efficient approach to unlock the potential of cell metabolism for fatty acid production in E. coli . Improving fatty acid production by tuning translation rates Engineering mutant and hybrid promoters with modified RNA polymerase, activator or repressor-binding activities has been widely used in metabolic engineering for transcriptional fine-tuning and pathway optimization [17] , [27] , [28] . However, the genetic recalcitrance of the bacteriophage T7 promoter has restricted our ability to manipulate the consensus promoter core sequence (−35 and −10 region) and the lacI repressor binding region ( lacO ) [29] . Instead, we opted to refine the translation initiation rate of both the GLY and FAS modules to further balance the supply of malonyl-CoA and consumption of malonyl-ACP in our expression system. The four RBSs, RBS 29–32, chosen from the MIT Registry of Biological Standard Parts, were used to replace the 5′-UTR region (5′-untranslated region) of the native T7 promoter ( Fig. 3a ). To test the functionality of engineered RBS variants, enhanced fluorescence protein was used as a reporter and the rate of fluorescence change normalized with cell density was used to characterize RBS activity ( Fig. 3b ). Results shown here indicate that the engineered RBSs showed differential translational activities ranging from 0.18 to 3 relative to RBS32. All the tested T7-RBS reporters exhibited the desirable on–off switching property with dynamic ranges spanning over four orders of magnitude in response to isopropyl-β- D -thiogalactoside (IPTG) ( Fig. 3b ), indicating the introduced RBS did not change the T7 promoter functionality. 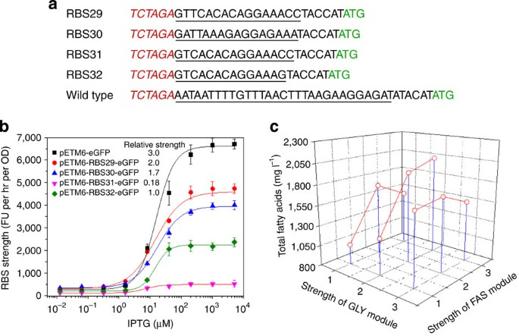Figure 3: Tuning translation initiation rate to improve fatty acid production. (a) Selected ribosome binding sites (RBSs) are from the MIT Registry of Standard Biological Parts. Underscored sequence is RBS core sequence; Italic red sequence showsXbaI site; start codon is shown in green colour. (b) The dose response of promoter activity to inducer IPTG using five versions of RBS harboured byE. coliBL21*(DE3) in Luria broth media at 30 °C. (c) Optimization of fatty acid production by balancing the RBS strength of GLY and FAS modules inmGLY-lACA-hFAS construct. GLY and FAS modules were expressed either under the control of a weak RBS (RBS32, relative strength 1), moderate RBS (RBS29, relative strength 2) or strong RBS (wild type, relative strength 3). All experiments were performed in triplicate and error bars show s.d. with 95% CI. Figure 3: Tuning translation initiation rate to improve fatty acid production. ( a ) Selected ribosome binding sites (RBSs) are from the MIT Registry of Standard Biological Parts. Underscored sequence is RBS core sequence; Italic red sequence shows Xba I site; start codon is shown in green colour. ( b ) The dose response of promoter activity to inducer IPTG using five versions of RBS harboured by E. coli BL21*(DE3) in Luria broth media at 30 °C. ( c ) Optimization of fatty acid production by balancing the RBS strength of GLY and FAS modules in m GLY- l ACA- h FAS construct. GLY and FAS modules were expressed either under the control of a weak RBS (RBS32, relative strength 1), moderate RBS (RBS29, relative strength 2) or strong RBS (wild type, relative strength 3). All experiments were performed in triplicate and error bars show s.d. with 95% CI. Full size image With the characterized RBSs, we set out to test whether variations of the 5′-UTR region in both the GLY and FAS modules would impact overall fatty acid production. By placing each of the module genes under the control of a strong (native RBS, relative strength 3), moderate (RBS29, relative strength 2) and weak (RBS32, relative strength 1) RBS, we combinatorially constructed nine strains to identify conditions that could optimize the expression of the GLY and FAS modules ( Fig. 3c ). As the downstream pathway (FAS module) expression increases from very low levels, fatty acid production also rises initially because of the increased driving force for conversion of malonyl-ACPs to the final products. Further increase in the FAS expression led to large disparities in fatty acid production, with maximal production achieved when upstream pathway (GLY module) was expressed from a moderate strength RBS. This inconsistency could partially be attributed to the metabolic imbalance associated with either depleted or accumulated acetyl-CoA flux due to the relatively low or high expression of GLY module. The optimized strain (rbs29- m GLY- l ACA- h FAS) resulted in a final volumetric production of 2.04 g l −1 of total fatty acids, representing an additional 46% increase compared with the parental strain ( m GLY- l ACA- h FAS, 1.4 g l −1 ). Fatty acids production under controlled culture conditions We next tested the fatty acid production of the optimized strains (rbs29- m GLY- l ACA- h FAS) in a fed-batch 20-L fermenter (working volume: 15 L). pH-Stat control and glucose feeding were started when the initial glucose (2%) was almost depleted and the dissolved oxygen showed a sharp increase ( Fig. 4a ). Glucose feeding was limited at a constant flow rate of 1.235 ml min −1 (0.494 g Glucose per min) to minimize the secretion of toxic byproduct acetic acid. Fermentation was ended after around 70 h of cultivation when all the 4.5 l of 40% glucose was exhausted. It was interesting to find that addition of 0.65 mM IPTG at 8 h of cultivation drove the cell to a diauxic growth pattern ( Fig. 4b ), accompanied with the slow uptake of oxygen. This diauxic growth to a large extent could be attributed to the adjustment of metabolism from cell growth for synthesizing recombinant proteins due to the induction of T7 RNA polymerase. After a long adaptation period (from 20 to 45 h), cells started to grow slowly with rapid glucose and oxygen consumption. The lower specific production rate in the second phase could be possibly attributed to the limited oxygen transfer and lower genetic stability of constructed pathways in BL21 strains ( Fig. 4a and Supplementary Fig. S6 ). At the end of the cultivation, the engineered strain (rbs29- m GLY- l ACA- h FAS) produced 8.6 g l −1 of free fatty acids from 110 g l −1 of glucose with a maximal dry cell density 40.86 g DCW l −1 (optical density was 90.8) and a productivity 0.124 g fatty acids h −1 l −1 , the highest production titre and productivity reported to date. 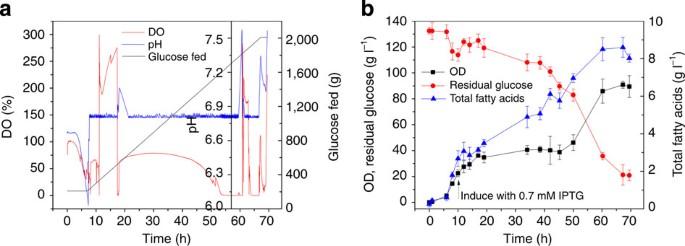Figure 4: Fed-batch cultivation of engineered strain in a 20-l bioreactor. (a) Time course of dissolved oxygen (DO), pH and the total glucose (in g) fed in the fermenter. Forty percentage glucose (w/w) was fed at a constant rate of 1.235 ml min-1. pH was maintained at 6.8 by a proportional-integral derivative (PID) controller by feeding 5 N ammonium hydroxide. DO was maintained by sparging the fermenter with air or pure oxygen. (b) Time course profile of cell growth (OD), net residual glucose and total fatty acid production of the strain BL21ΔfadDexpressing pCDM4-[RBS29]-GLY, pACM4-ACA and pETM6-FAS in 20-l bioreactor. Net residual glucose was calculated based on the difference between the total amount of glucose fed and the instantaneous glucose left. Fermentation assays were performed in duplicate and error bars show s.d. with 95% CI. Figure 4: Fed-batch cultivation of engineered strain in a 20-l bioreactor. ( a ) Time course of dissolved oxygen (DO), pH and the total glucose (in g) fed in the fermenter. Forty percentage glucose (w/w) was fed at a constant rate of 1.235 ml min -1 . pH was maintained at 6.8 by a proportional-integral derivative (PID) controller by feeding 5 N ammonium hydroxide. DO was maintained by sparging the fermenter with air or pure oxygen. ( b ) Time course profile of cell growth (OD), net residual glucose and total fatty acid production of the strain BL21Δ fadD expressing pCDM4-[RBS29]-GLY, pACM4-ACA and pETM6-FAS in 20-l bioreactor. Net residual glucose was calculated based on the difference between the total amount of glucose fed and the instantaneous glucose left. Fermentation assays were performed in duplicate and error bars show s.d. with 95% CI. Full size image Early metabolic engineering studies on fatty acid production have been dedicated to optimizing precursor supply and the specificity of plant fatty acyl-ACP thioesterase [4] , [6] , [10] , [30] , [31] . Engineering the reversal of β-oxidation pathway [7] and a dynamic sensor-regulator system [32] have also led to the production of fatty-acid-derived long chain chemicals and fuels. Despite these achievements, further improvement in fatty acid production requires systematic investigation of pathway limitations and removing metabolic constraints that are intrinsic to the tightly regulated cell metabolism. As a result, a number of synthetic biology approaches have been proposed to balance the precursor flux distribution including modification of plasmid copy number [33] , promoter strength [34] and gene codon usage [12] . However, most of these approaches are not modular and require time-consuming work tweaking the individual pathway components until the desired performance is achieved, which greatly compromises our ability to exploit the full potential of cell metabolism. Here we demonstrate that E. coli central carbon metabolism can be leveraged to produce large quantities of fatty acids, which potentially could be used as renewable fuel alternatives. Elimination of the fatty acid degradation pathway by deletion of fatty acyl-CoA synthetase ( fadD ) along with the boosting of rate-limiting precursor (malonyl-CoA) flux by the expression of the four subunit acetyl-CoA carboxylase ( accaABCD ) led to a strain producing three-fold more fatty acids. To relieve the feedback inhibition of β-ketoacyl-ACP synthase ( fabB or fabH ) caused by the accumulation of fatty acyl-ACPs [23] , E. coli multifunctional fatty acyl-CoA thioesterase (truncated tesA′ ) and three plant fatty acyl-ACP thioesterases ( BnFatA , CnFatB2 and EgTE ) were expressed to convert fatty acyl-ACPs into fatty acids and terminate the chain elongation cycle. Interestingly, the composition and chain length of fatty acids can be controlled by expressing different thioesterases, with the native thioesterase ( tesA′ ) producing up to 27.8% of medium chain myristic acid and fatB2 from C . nucifera producing up to 55.3% palmitic acid ( Supplementary Fig. S2 ). Consistent with previous studies, fatty acyl-ACP thioesterase has been identified as the major determinant of the chain length and level of saturated fatty acids in plants [35] . Tailor-made derivatives of such medium chain fatty acids could potentially be used as jet fuel supplements due to their extremely low freezing point and high energy density [36] . In addition to malonyl-CoA, acetyl-CoA has also previously been identified as a rate-limiting step for producing a range of recombinant compounds including polyketides [21] and flavonoids [20] . Boosting acetyl-CoA flux by overexpressing parts of the glycolytic pathway significantly improved fatty acid production. But co-overexpression of the glycolysis pathway and fatty acid synthesis pathway led to a suboptimal production, pointing out a metabolic imbalance between the production of acetyl-CoA and its subsequent conversion to malonyl-CoA and fatty acids. This led us to partition the E. coli central metabolic network into three modules: the acetyl-CoA formation module (GLY encoded by pgk , gapA , aceE , aceF and lpdA ), acetyl-CoA activation module (ACA encoded by accABCD and fabD ), and malonyl-ACP consumption module (FAS encoded by fabAHGI and CnfatB2 ). To unleash the E. coli metabolic potential, multivariate modular pathway engineering that focuses on optimizing the expression of these three modules was employed, and yielded a 20-fold increase in fatty acid production from shake-flask cultures. Further pathway engineering was targeted at tuning the translational efficiency of the precursor pathway and fatty acids synthesis pathway, as several studies have shown that protein translation efficiency is largely dependent on the 5′-UTR and RBS region [37] , [38] . Expression of acetyl-CoA-producing pathway (GLY module) and malonyl-ACP-consuming pathway (FAS module) was balanced by combinatorially altering the strength of RBSs of both GLY and FAS modules. Production potential of the optimal strain was tested in a 20-l fed-batch fermenter with constant glucose feeding and a final titre of 8.6 g l −1 total fatty acids was obtained with a productivity of 0.124 g fatty acids h −1 l −1 . As a promising alternative fuel source, the high yield of free fatty acids achieved in this study may provide an economically feasible process for producing fatty acid-derivatized fuels. In addition, the multivariate modular strategies used in this study should be directly applicable to engineering microbial production of other valuable metabolites, especially ones derived from malonyl-CoA and acetyl-CoA. FAS module construction Pathway construction and DNA manipulations were performed following standard molecular cloning protocols. Strains and plasmids used in this study are listed in Supplementary Table S1 . All PCR primers used for chromosomal gene inactivation, gene amplification and site-directed mutagenesis are listed in Supplementary Table S2 . Detailed pathway construction procedure including gene deletion, GLY module, ACA module and GLY/FAS module with RBS variants is described in the Supplementary Methods . Brassica napus fatty acyl-ACP thioesterase BnfatA (Gene ID: X73850.1), C. nucifera fatty acyl-ACP thioesterase CnfatB2 (Gene ID: JF338904.1), Elaeis guineensis fatty acyl-ACP thioesterase EGTE (Gene ID: AF110462.1) and E. coli β-ketoacyl-ACP synthase III fabH (Ecocyc Accession Numbers: EG10277) were codon-optimized and synthesized by GenScript. Detailed sequence information is provided in Supplementary Table S3 . BnFatA, CnFatB2, EGTE and fabH were subcloned into pETM6 to give pETM6-BnFatA, pETM6-CnFatB2, pETM6-EGTE and pETM6-fabH, respectively. E. coli β-hydroxy acyl-ACP dehydrase fabA , β-ketoacyl-ACP reductase fabG , enol acyl-ACP reductase fabI and multifunctional thioesterase tesA ′ gene fragments were PCR amplified from E. coli K-12 genomic DNA using primer pairs FabA_NdF/FabA_XhR, FabG_NdF/FabG_XhR, FabI_NdF/FabI_XhR and tesA′_NdF/tesA′_XhR, respectively. Nde I/ Xho I-digested PCR fragments were ligated to the Nde I and Xho I-digested pETM6 to give constructs pETM6-fabA, pETM6-fabG, pETM6- fabI and pETM6-tesA′, respectively. ePathBrick-directed gene assembly was performed based on these individual constructs [26] . Briefly, pseudo-operon configuration was achieved by ligating the Avr II/ Sal I-digested donor construct with the Spe I/ Sal I-digested receiver construct. Multi-fragment assembly can be performed in parallel and in rare cases, high affinity Apa I site on lacI gene was used (instead of Sal I) to balance the insertion and vector size, and therefore improve the ligation efficiency. Iterative assembly was performed and the final construct pETM6-CnFatB2-fabAHGI was named pETM6-FAS. The large fragment of Avr II and Sal I-digested pETM6-FAS was ligated to the Avr II and Sal I-digested pACM4, pCDM4, pCOM4 and pRSM3 to give constructs pACM4-FAS, pCDM4-FAS, pCOM4-FAS and pRSM3-FAS, respectively. All constructs were screened by restriction enzyme digestion and verified by gene sequencing. Fatty acid fed-batch fermentation A detailed fermentation procedure of the fatty acids shake-flask experiments can be found in the Supplementary files. For 20-l fed-batch fermentation, strain BL21(DE3) Δ fadD with pCDM4-[RBS29]-GLY, pACM4-ACA and pETM6-FAS was used to test the fatty acid production potential. Frozen stocks were used to inoculate 10 ml MK media (13.5 g l −1 KH 2 PO 4 , 4.0 g l −1 (NH 4 ) 2 HPO 4 , 1.7 g l −1 citric acid, 20 g l −1 glucose and 10 g l −1 yeast extract, 10 ml l −1 trace metals and pH adjusted to 6.8 by sodium hydroxide) with appropriate antibiotics in 50 ml corning tubes and allowed to grow at 37 °C for 12 h. Trace metal solution consisted of (per liter of 5 M HCl) 10.0 g FeSO 4 ·7H 2 O, 2.0 g CaCl 2 , 2.2 g ZnSO 4 ·7H 2 O, 0.5 g MnSO 4 ·4H 2 O, 1.0 g CuSO 4 ·5H 2 O, 0.1 g (NH 4 ) 6 Mo 7 O 24 ·4H 2 O and 0.02 g Na 2 B 4 O 7 ·10H 2 O (ref. 39 ). Ten milliliter of seed culture was inoculated to 200 ml MK media (pH 6.8, with trace metal and appropriate antibiotics) and grown at 37 °C for 6 h. Then 400 ml of seed culture was used to inoculate 9.6 l MK media (pH 6.8, with trace metal and appropriate antibiotics) in a 20 l BioFlo4500 Bioreactor (New Brunswick). The bioreactor was controlled at batch mode in the first 8 h and then switched to fed-batch mode by feeding 5 N ammonium hydroxide and 40% glucose (w/w). pH was maintained at 6.8 by feeding NH 4 OH and glucose was fed at a constant flow rate of 1.235 ml min −1 with two independently controlled peristaltic pumps. Induction of protein expression was performed by adding 2.4 g IPTG and switching the cultivation temperature to 34 °C at 8 h of fermentation (OD=13). Dissolved oxygen, pH and the amount of glucose fed were collected every 10 s using a BioCommand software. Samples were taken every 4–6 h to measure cell density, fatty acid production and residual glucose level. Fatty acid extraction and analytical procedure Free fatty acids were extracted following a modified protocol as described by Voelker [40] . Detailed extraction protocol is described in the Supplementary Methods . For quantification, both intracellular and extracellular fatty acids were analysed by GC–MS. For HPLC analysis, crude fatty acids were mixed with 150 μl of 10 mg ml −1 triethylamine (wt/v, acetone solution) and 150 μl 10 mg ml −1 phenacyl bromide (wt/v, acetone solution). The reaction mixture was incubated in a 50 °C water bath for 4 h. Using pentadecanoic acid as an internal standard, the resulting fatty acid phenacyl esters were analysed at 254 nm by an Agilent 1260 HPLC system [41] equipped with a ZORBAX SB-C18 column (5 μm, 4.6 × 150 mm) kept at 25 °C and a diode array detector. The elution profile was 0–5 min with 35% acetonitrile (ACN), 6–10 min with 50% ACN, 11–14 min with 85% ACN and 15–25 min with 100% ACN. For GC–MS analysis, crude fatty acids were re-dissolved in 300 μl 5% (vol/vol) H 2 SO 4 in methanol, and incubated in a sealed vial at 80 °C for 4 h. A total of 300 μl 0.9% (wt/vol) NaCl was added to the reaction mixture and the resulting fatty acid methyl esters were extracted with 200 μl of n -hexane. Overall, 1.5 μl of the hexane layer was directly injected to a Shimadzu QP5050-Quadrupole Gas Chromatograph-Mass Spectrometer for analysis. The temperature profile was 60 °C for 2.5 min, ramp at a rate of 20 °C min −1 to 250 °C, ramp at a rate of 10 °C min −1 to 325 °C and hold at 325 °C for 5.5 min. Injection temperature was set at 250 °C and MS scan speed was 2,000 μ sec −1 . GC column was Agilent DB-5 ms with film thickness 0.25 μm, diameter 0.25 mm and length 30 m. Residual glucose was analysed by an Agilent 1260 HPLC system equipped with a ZORBAX Carbohydrate column (5 μm, 4.6 × 150 mm) kept at 30 °C and a refractive index detector (Agilent RID 1260). The mobile phase contained 50% ACN and 50% water with a flow rate of 1 ml min −1 . Samples were centrifuged at 12 000 r.p.m. for 3 min, and 10 μl of supernatant was directly injected to HPLC for analysis. The retention time for glucose was around 2.7 min. Nile red-based fatty acid quantification procedure is described in the Supplementary Methods . How to cite this article: Xu P et al . Modular optimization of multi-gene pathways for fatty acids production in E. coli . Nat. Commun. 4:1409 doi: 10.1038/ncomms2425 (2013).